The cytoplasmic coiled-coil mediates cooperative gating temperature sensitivity in the voltage-gated H+channel Hv1 Hv1/VSOP is a dimeric voltage-gated H + channel in which the gating of one subunit is reportedly coupled to that of the other subunit within the dimer. The molecular basis for dimer formation and intersubunit coupling, however, remains unknown. Here we show that the carboxy terminus ends downstream of the S4 voltage-sensor helix twist in a dimer coiled-coil architecture, which mediates cooperative gating. We also show that the temperature-dependent activation of H + current through Hv1/VSOP is regulated by thermostability of the coiled-coil domain, and that this regulation is altered by mutation of the linker between S4 and the coiled-coil. Cooperative gating within the dimer is also dependent on the linker structure, which circular dichroism spectrum analysis suggests is α-helical. Our results indicate that the cytoplasmic coiled-coil strands form continuous α-helices with S4 and mediate cooperative gating to adjust the range of temperatures over which Hv1/VSOP operates. Hv1/VSOP is a recently discovered voltage-gated H + channel (Hv) [1] , [2] that is expressed in immunocytes and is involved in the production of reactive oxygen species in phagocytes [3] , [4] , [5] and the antigen response in B lymphocytes [6] . Hv1/VSOP has four-transmembrane segments that correspond to the voltage-sensor domain (S1-S4) of other voltage-gated channels [1] , [2] , it does not have a canonical pore domain, and the voltage-sensor domain is thought to act as both the voltage-sensor and the H + -permeation pathway [7] . The composition of the functional unit by the minimally designed voltage-gated channel subunit is dimeric [8] , [9] , [10] . Most types of ion channels have oligomeric architectures. In the case of the voltage-gated K + channel (Kv), electrophysiological studies with toxin blockers showed the functional unit to be a tetramer [11] , a finding that was confirmed by X-ray crystallography [12] , [13] , [14] , [15] . Assembly of the four subunits into the tetrameric channel forms the permeation pathway in the centre. In the Hv channel, by contrast, only one subunit of the dimeric functional unit is sufficient for its channel activity [8] , [10] . The functional role of dimer formation, hence, lies outside the formation of the permeation pathway. One characteristic derived from the dimer assembly in the Hv channel is the cooperative channel gating—that is, the gating movement of one monomeric channel subunit affects the gating of the other subunit within the dimeric unit [16] , [17] , [18] . However, it remains unclear through which part of the channel the conformational change is transmitted from one subunit to the other during channel gating. A certain level of physical intersubunit contact between transmembrane regions has been shown by biochemical approaches [9] , raising the possibility that the cooperative gating in the dimer is mediated via interaction between the tramsmembrane domains. Meanwhile, Hv1/VSOP contains a conserved coiled-coil motif in the cytoplasmic region. The dimeric structure of the carboxy terminus cytoplasmic coiled-coil domain of the human Hv1/VSOP was analysed recently [19] . This indicates that the Hv channel has an intersubunit contact in the cytoplasmic region. However, the roles of the coiled-coil domain in the function of Hv channels remain unclear. One possibility for the significance of the coiled-coil is that it is required for situating two monomers close to each other and provides just a platform for a physical interaction between two monomers in the membrane. The other possibility is that the conformational change of one subunit is transmitted to the other by the cytoplasmic coiled-coil, and the structural features and the chemical properties of the coiled-coil domain make significant contributions to channel gating. To address this issue and to investigate the significance of dimerization, we analyse the relationship between dimer formation and channel gating in the mouse Hv channel (mHv1/VSOP) using X-ray crystallography, circular dichroism (CD) spectroscopy and electrophysiology. We find that dimer formation and cooperative gating in mHv1/VSOP are mediated via the cytoplasmic domain. We also find that this mechanical interaction by the dimeric assembly unit was wrought by an uninterrupted helical structure from S4 to the coiled-coil region. Coiled-coil assembly domain of mHv1/VSOP and its structure Hv1/VSOP is a minimal voltage-gated ion channel that has only four transmembrane regions (S1-S4), which comprise a voltage-sensor domain [1] , [2] . In addition, a C-terminal cytoplasmic domain consisting of ~55 residues is well conserved among species ( Fig. 1a ). Beginning ~10 residues C-terminal to the last transmembrane domain (S4), there is a distinctive heptad repeat pattern (abcdefg) n characteristic of a coiled-coil architecture, in which the 'a' and 'd' positions are hydrophobic amino acids and other positions are hydrophilic ( Fig. 1a ; Supplementary Fig. S2a ). 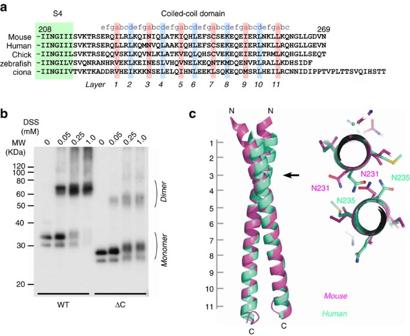Figure 1: Determination and structure comparison of the coiled-coil assembly domain. (a) Sequence alignment of the C-terminal cytoplasmic coiled-coil domain of Hv channel from various species. The positions of the coiled-coil heptad repeat (abcdefg) are indicated above the alignment. Coiled-coil residues occupying hydrophobic 'a' and 'd' positions are denoted by blue and red, respectively. Layer positions for each residue in the structure are indicated below the alignment. The green box depicts part of S4. (b) Oligomeric state of mHv1/VSOP channels studied by crosslinker analysis with western blotting. WT and C-terminus-truncated (ΔC) mHv1/VSOPs were expressed in HEK293 cells and treated with the indicated concentrations of DSS. (c) Comparison of the coiled-coil domain between mHv1/VSOP (violet) and hHv1/VSOP (green, PDB code: 3A2A). Two cartoon helix models are superimposed. Layer numbers and the N- and C-termini of the coiled-coil are indicated. The overall r.m.s. deviation of Cα atoms of each molecules (residues 222–262 of mouse versus 226–266 of human) is 0.798 Å, and that of the C-terminal half of the coiled-coil (235–262 of mouse versus 239–266 of human) is 0.377 Å. Right panel indicates the comparison of Asn in layer-3 between mHv1/VSOP (violet) and hHv1/VSOP (green) coiled-coils. Two structures (shown as stick and cartoon helix models) are superimposed. In hHv1/VSOP, the residue corresponding to N231 in mHv1/VSOP is N235. Figure 1: Determination and structure comparison of the coiled-coil assembly domain. ( a ) Sequence alignment of the C-terminal cytoplasmic coiled-coil domain of Hv channel from various species. The positions of the coiled-coil heptad repeat (abcdefg) are indicated above the alignment. Coiled-coil residues occupying hydrophobic 'a' and 'd' positions are denoted by blue and red, respectively. Layer positions for each residue in the structure are indicated below the alignment. The green box depicts part of S4. ( b ) Oligomeric state of mHv1/VSOP channels studied by crosslinker analysis with western blotting. WT and C-terminus-truncated (ΔC) mHv1/VSOPs were expressed in HEK293 cells and treated with the indicated concentrations of DSS. ( c ) Comparison of the coiled-coil domain between mHv1/VSOP (violet) and hHv1/VSOP (green, PDB code: 3A2A). Two cartoon helix models are superimposed. Layer numbers and the N- and C-termini of the coiled-coil are indicated. The overall r.m.s. deviation of Cα atoms of each molecules (residues 222–262 of mouse versus 226–266 of human) is 0.798 Å, and that of the C-terminal half of the coiled-coil (235–262 of mouse versus 239–266 of human) is 0.377 Å. Right panel indicates the comparison of Asn in layer-3 between mHv1/VSOP (violet) and hHv1/VSOP (green) coiled-coils. Two structures (shown as stick and cartoon helix models) are superimposed. In hHv1/VSOP, the residue corresponding to N231 in mHv1/VSOP is N235. Full size image To verify that the C-terminal cytoplasmic domain is required for formation of the Hv channel dimer, crosslinking assays were performed on the mouse Hv1/VSOP (mHv1/VSOP) expressed in HEK293 cells. In full-length mHv1/VSOP, a twofold molecular weight on SDS–PAGE was observed with disuccinimidyl suberate (DSS) ( Fig. 1b ) [10] , confirming that mHv1/VSOP is expressed as a dimer. Deletion of the C-terminal domain (ΔC) remarkably reduced the dimer fraction ( Fig. 1b ). Sedimentation equilibrium experiments showed that the C-terminal domain of mHv1/VSOP protein forms dimer in solution ( Supplementary Fig. S1a ). 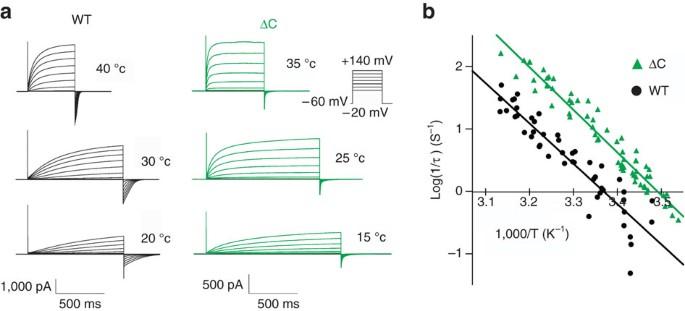Figure 2: Effect on the activation kinetics by deletion of the coiled-coil domain. (a) Representative currents through WT (black) and ΔC (green) mHv1/VSOP recorded at the indicated temperatures from HEK293 cells. The holding potential was −60 mV; step pulses from −20 mV to +140 mV were applied in 20-mV increments. The pulse protocol is indicated in the right. (b) Accumulated data from WT (black) and ΔC (green) channels and the linear regression lines showing the correlation of the activation kinetics with temperature. Figure 2: Effect on the activation kinetics by deletion of the coiled-coil domain. ( a ) Representative currents through WT (black) and ΔC (green) mHv1/VSOP recorded at the indicated temperatures from HEK293 cells. The holding potential was −60 mV; step pulses from −20 mV to +140 mV were applied in 20-mV increments. The pulse protocol is indicated in the right. ( b ) Accumulated data from WT (black) and ΔC (green) channels and the linear regression lines showing the correlation of the activation kinetics with temperature. Full size image To determine the biochemical characteristics of the coiled-coil of mHv1/VSOP, we solved a crystal structure of the coiled-coil domain (mHv1/VSOP-cc, residues 220–269), and compared it with the human Hv1/VSOP (hHv1/VSOP) coiled-coil [19] . The amino terminus of the mHv1/VSOP coiled-coil is bent and deviates from the hHv1/VSOP structure ( Fig. 1c ). The coiled-coil core consists largely of well-packed hydrophobic residues. In the centre of the N-terminal half, hydrophilic Asn residues (N231), instead of hydrophobic residues, comprise the core at layer 3 ( Fig. 1c ). They are asymmetrically packed, and, notably, the side-chain of N231 shows a flipped geometry in comparison with the hHv1/VSOP structure ( Fig. 1c ). The neighbouring residues, at positions 'g' and 'b', are unusually hydrophobic (I230 and I232) ( Fig. 1a ; Supplementary Fig. S2a ). Given the reports from the GCN4 coiled-coil, a yeast leucine zipper protein [20] , [21] , [22] , the hydrophilic core residues, N231, could be a weakness of the core packing stability. Other structure features are the lack of inter-subunit polar interaction that stabilizes the assembly [23] , [24] , [25] ( Supplementary Fig. S2b ) and the dual-conformation of Cys residues in the core, suggesting a possibility of switching of the disulfide bonding in response to redox ( Supplementary Fig. S2c ). The temperature dependence of the CD signal of mHv1/VSOP-cc shows a cooperative loss of structure ( Fig. 3d and Supplementary Fig. S1b ), consistent with a well-folded complex having an extensive hydrophobic core. The melting temperature (apparent Tm= 40.6, 40.8 °C ( n =2)) was lower than those of other naturally occurring coiled-coil proteins (Tm>60 °C) [26] , [27] , [28] , [29] , and unfolding of the mHv1/VSOP-cc coiled-coil was irreversible ( Fig. 3d ). Thus, the mHv1/VSOP assembles into a dimer using a cytoplasmic dimer coiled-coil architecture that is a well-folded and thermally labile coiled-coil. Structure details and comparisons with hHv1/VSOP are summarized in Supplementary Fig. S2 . 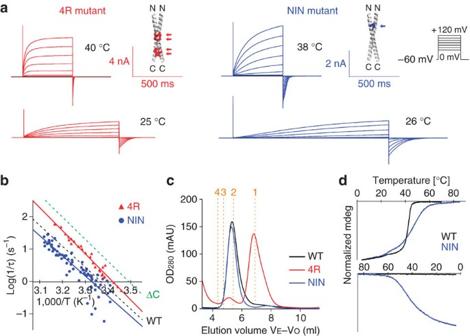Figure 3: The activation kinetics of coiled-coil mutant channels. (a) Representative currents through 4R (red) and NIN (blue) mHv1/VSOP recorded at the indicated temperatures from HEK293 cells. The pulse protocol is indicated in the right. Arrows point positions of the mutations. (b) Accumulated data from 4R (red) and NIN (blue) mutant channels and the linear regression lines. Symbols used are shown in the figure. Dotted lines depict the linear regression lines. (c) Coiled-coil stoichiometry determined by Superdex 200 (GE Healthcare) size-exclusion chromatography monitored at 280 nm. For clear-size separation, we used HMT-tagged mHv1/VSOP-cc proteins in these experiments. The horizontal axis shows elution volume (ml), and dotted lines indicate the predicted elution volumes for tetrameric, trimeric, dimeric and monomeric proteins. The elution volumeVEwas corrected for the void elution volume (VO). Molecular weights were calculated using standard curves (Supplementary Fig. S9). Oligomeric state of the main component was 2.29±0.01 (n=3) for WT, 1.15±0.05 (n=3) for 4R and 2.35±0.05 (n=3) for NIN. (d) Temperature dependence of the CD signal recorded from mHv1/VSOP-cc WT and NIN mutant proteins at 222 nm. Signals were recorded while applying a heating (top) or cooling (bottom) temperature gradient. Figure 3: The activation kinetics of coiled-coil mutant channels. ( a ) Representative currents through 4R (red) and NIN (blue) mHv1/VSOP recorded at the indicated temperatures from HEK293 cells. The pulse protocol is indicated in the right. Arrows point positions of the mutations. ( b ) Accumulated data from 4R (red) and NIN (blue) mutant channels and the linear regression lines. Symbols used are shown in the figure. Dotted lines depict the linear regression lines. ( c ) Coiled-coil stoichiometry determined by Superdex 200 (GE Healthcare) size-exclusion chromatography monitored at 280 nm. For clear-size separation, we used HMT-tagged mHv1/VSOP-cc proteins in these experiments. The horizontal axis shows elution volume (ml), and dotted lines indicate the predicted elution volumes for tetrameric, trimeric, dimeric and monomeric proteins. The elution volume V E was corrected for the void elution volume ( V O ). Molecular weights were calculated using standard curves ( Supplementary Fig. S9 ). Oligomeric state of the main component was 2.29±0.01 ( n =3) for WT, 1.15±0.05 ( n =3) for 4R and 2.35±0.05 ( n =3) for NIN. ( d ) Temperature dependence of the CD signal recorded from mHv1/VSOP-cc WT and NIN mutant proteins at 222 nm. Signals were recorded while applying a heating (top) or cooling (bottom) temperature gradient. Full size image Thermostability of the coiled-coil and the channel gating We assessed the functional significance of dimeric coiled-coil assembly in the mHv1/VSOP, using whole-cell patch clamp recordings. Deletion of the C-terminal coiled-coil domain accelerated the channel's activation kinetics ( Fig. 2a ). The activation kinetics reflect the transition between the open and closed states of the channel and are temperature-dependent, and, given that the assembly of the mHv1/VSOP coiled-coil was thermally labile ( Fig. 3d ; Supplementary Fig. S1b ), we analysed the relationship between temperature and activation kinetics. We found that the activation kinetics of the full-length channel at 40 °C was similar to that of ΔC at 25 °C, while activation of the full-length channel at 30 °C was similar to that of ΔC at 15 °C ( Fig. 2a ). Thus deletion of the coiled-coil domain shifted the thermosensitivity relationship by 15 °C without changing the slope ( Fig. 2b ). In the analyses of the temperature-dependent activation, we confirmed that the kinetics was not dependent on the current amplitude but highly dependent on the recording temperature ( Supplementary Figs S3a,b ). We also analysed the effect of the pre-heating for the activation kinetics, and activation kinetics were little changed by the preheating ( Supplementary Fig. S3c ). We next tested the effects of introducing mutations that disrupt the coiled-coil. Bulky hydrophilic Arg residues were introduced into the well-packed hydrophobic core layers in the C-terminal half of the coiled-coil (layers 5, 6, 9 and 10 in Fig. 1c and Supplementary Fig. S2a ). This '4R' mutation accelerated the channel's activation kinetics to some extent ( Fig. 3a), and shifted the thermosensitivity relationship by ~8 °C in the direction of the ΔC phenotype ( Fig. 3b ). We also confirmed that assembly of the dimeric coiled-coil domain was suppressed in the 4R mutant as shown by size exclusion chromatography ( Fig. 3c ). On the other hand, to stabilize the coiled-coil assembly, we introduced an inverse mutation, NIN, into the amino-acids sequence at INI (230–232), where the NIN mutation makes the periodic hydrophobicity more complete in the heptad-repeat of the coiled-coil protein [21] . The NIN mutation showed a slower activation ( Fig. 3a ) and shifted the thermosensitivity relationship by ~5 °C away from the wild-type (WT) phenotype ( Fig. 3b ). In the CD spectrum of the coiled-coil protein, the coiled-coil folding became reversible ( Fig. 3d ; Supplementary Fig. S1c ). The melting was non-sigmoidal, suggesting that the melting occurs in a more complex manner than a simple two-state transition ( Fig. 3d ). These results suggest that the characteristics of the coiled-coil assembly were altered and stabilized by the NIN mutation. The single-point mutation, N231L, did not lead to a clear change in the activation kinetics, suggesting that the surrounding residues, I230 and I232, also contribute to the stability of the coiled-coil ( Supplementary Fig. S4 ). We also confirmed that NIN mutation did not change the dimer stoichiometry ( Fig. 3c ). Taken together, the stability of the C-terminal domain determined the channel activation kinetics in a temperature-dependent manner such that coiled-coil dimer assembly inhibited channel activation. Importance of the linker in the temperature-dependent gating The ΔC channel retains a monomeric form ( Fig. 1b ), whereas the WT channel assembles as a dimeric channel and the gating showed higher thermostability ( Fig. 2a,b ). Suppression of the dimerization by 4R mutation destabilized the thermostability of the gating ( Fig. 3a,b ). One interpretation for these results could be that the mere dimerization of the channel can lead to thermostability of the gating by spacing two monomers in close proximity. To test this idea, we made two types of concatenated channel harbouring/lacking the coiled-coil domain (Tandem/ΔC-Tandem) and analysed their activation ( Fig. 4a , illustration). The Tandem channel showed similar activation kinetics to WT ( Fig. 4a ). On the other hand, the ΔC-Tandem channel showed faster activation kinetics than WT, and the thermosensitivity relationship was indistinguishable from that of the ΔC phenotype ( Fig. 4a ). We also confirmed that both of the N-terminal and the C-terminal subunit in the ΔC-Tandem channel are intact in function ( Supplementary Fig. S5 ). These results suggest that the mere positional proximity of two channels is not sufficient to produce the thermal stability in the WT phenotype, and the coiled-coil domain is necessary. 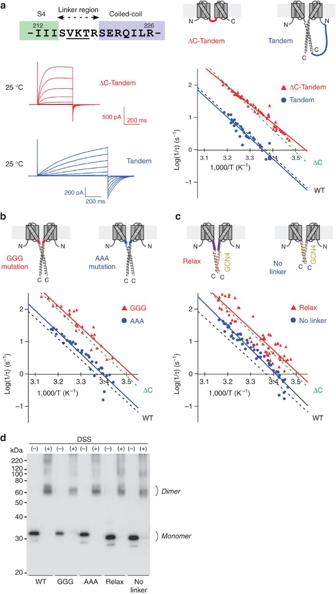Figure 4: Temperature-dependent activation of linker mutant channels. (a) Amino-acid sequence of linker residues between the coiled-coil domain and the last transmembrane domain (S4) (upper panel). Three residues, VKT, mutated to GGG/AAA in (b) are underlined. Representative currents through Tandem (blue) and ΔC-Tandem (red) channels recorded at 25 °C from HEK293 cells (lower panel). Accumulated data from the Tandem (blue) and the ΔC-Tandem (red) channels and the linear regression line (right panel) are shown; the dotted lines depict the linear regression lines for the data from WT (black) and ΔC (green) channels. (b) Accumulated data from the GGG (red) and AAA (blue) mutant channels and their linear regression lines; the dotted lines are the same as in panel (a). (c) Accumulated data from the GCN4 chimeric channel with a long linker (relax) (red) or with no linker (blue) and their linear regression lines; the dotted lines are the same as in panel (a). (d) Oligomeric state analysis of the mutant channels determined by crosslinker analysis with western blotting. mHv1/VSOP WT, the GGG and AAA mutants, and the relax and no linker chimeras were expressed in HEK293 cell and treated with or without 1 mM DSS. Proteins were separated on SDS–PAGE and immunoblotted with anti-mHv1/VSOP antibody. Figure 4: Temperature-dependent activation of linker mutant channels. ( a ) Amino-acid sequence of linker residues between the coiled-coil domain and the last transmembrane domain (S4) (upper panel). Three residues, VKT, mutated to GGG/AAA in ( b ) are underlined. Representative currents through Tandem (blue) and ΔC-Tandem (red) channels recorded at 25 °C from HEK293 cells (lower panel). Accumulated data from the Tandem (blue) and the ΔC-Tandem (red) channels and the linear regression line (right panel) are shown; the dotted lines depict the linear regression lines for the data from WT (black) and ΔC (green) channels. ( b ) Accumulated data from the GGG (red) and AAA (blue) mutant channels and their linear regression lines; the dotted lines are the same as in panel ( a ). ( c ) Accumulated data from the GCN4 chimeric channel with a long linker (relax) (red) or with no linker (blue) and their linear regression lines; the dotted lines are the same as in panel ( a ). ( d ) Oligomeric state analysis of the mutant channels determined by crosslinker analysis with western blotting. mHv1/VSOP WT, the GGG and AAA mutants, and the relax and no linker chimeras were expressed in HEK293 cell and treated with or without 1 mM DSS. Proteins were separated on SDS–PAGE and immunoblotted with anti-mHv1/VSOP antibody. Full size image The coiled-coil structure that we characterized begins only five residues, Ser 215 -Val 216 -Lys 217 -Thr 218 -Arg 219 (linker region, Fig. 4a ), downstream of the last transmembrane helix. The last transmembrane helix corresponds to the S4 of voltage-gated channels and is known to move substantially when the channel opens [30] , [31] . It is possible that the ΔC-Tandem channel lost proper strand orientation for dimer interaction, thereby failing to show the wild-type dimer phenotype. We therefore examined the activation kinetics of mutants whose linker sequences were altered by substituting three residues in the linker sequence, Val-Leu-Thr (underlined in Fig. 4a ), with Gly-Gly-Gly or Ala-Ala-Ala. The thermosensitivity relationship of the GGG mutant showed the ΔC phenotype, while that of the AAA mutant showed the WT phenotype ( Fig. 4b ). This suggests that linker flexibility/stability affects the channel gating. We also tested chimeric channels harbouring the stable coiled-coil from GCN4, a yeast leucine zipper type transcription factor protein [20] . The thermosensitivity relationship of a GCN4 chimera with a six amino-acid linker (designated 'relax') showed the ΔC phenotype, while that of a GCN4 chimera without intervening linker sequence showed the WT phenotype ( Fig. 4b ). To verify that these mutant channels were expressed as dimers, crosslinking assay with western blotting was performed ( Fig. 4d ). All mutants and chimeras exhibited clear band shifts to a region corresponding to the molecular mass of dimer ( Fig. 4d ). It is reported that the cytoplasmic end of S4 helix is close to each other within a dimer, where Cys introduced into the position of Thr222 in hHv1/VSOP make a disulfide bond between two monomers [9] . To examine whether this spatial proximity was disarranged by the GGG mutation, we performed crosslinking experiments by oxidation with the T218C mHv1/VSOP mutants that corresponds toT222C in hHv1/VSOP. Both of the T218C and the 'GGG+T218C' mutants maintained the phenotypes in function regardless of the oxidation ( Fig. 5b,c ). They produced substantial amount of dimeric fractions by disulfide bondings ( Fig. 5d ), suggesting that the GGG mutation, which alters the functional phenotype, maintains a spatial proximity of two S4 helixes in the cytoplasmic end. We found that S215, three-residue upstream of T218 ( Fig. 5a ), is another closely opposite site that can be crosslinked by oxidation when it is replaced by Cys. S215C mutant also showed similar results as shown in the 'GGG+T218C' mutant ( Fig. 5b and d ). Almost no disulfide bonding was observed in the 'ΔC+T218C' channel ( Fig. 5d ), because this channel lacks coiled-coil domain that is indispensable for dimerization ( Fig. 1b ). Taken together, these results indicate that the close positioning of two channel subunits, bound by the coiled-coil domain, is not enough to acquire the thermal stability of the channel gating, but the linker stability between the coiled-coil domain and the transmembrane region is required. 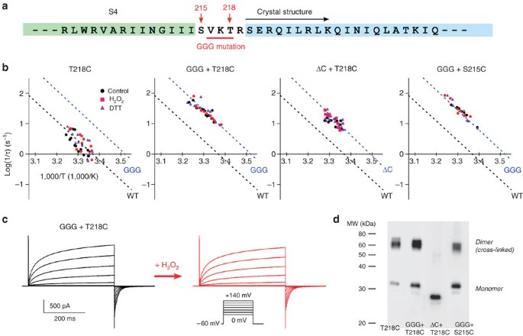Figure 5: Crosslinking analyses by oxidation in the cytoplasmic end of S4. (a) Schematic illustration of the mutation sites of S215, T218 and the GGG mutation. Constructs' designs were summarized in theSupplementary Fig. S9e. (b) Activation kinetics of the Cys-mutant channels were analysed under the control of temperature with the incubation of 5 mM H2O2(extracellular) or 1 mM DTT (in the pipette) for 15 min . The linear regression lines for the data from WT (black), GGG (blue) and ΔC (blue) channels were indicated. (c) Representative current traces of the GGG+T218C mutant channel before (black, left) and after (red, right) the incubation with H2O2. (d) Crosslinking western blot analyses with the oxidation for the Cys-mutant channels. Proteins did not migrate as dimers with reduction (not shown). Figure 5: Crosslinking analyses by oxidation in the cytoplasmic end of S4. ( a ) Schematic illustration of the mutation sites of S215, T218 and the GGG mutation. Constructs' designs were summarized in the Supplementary Fig. S9e . ( b ) Activation kinetics of the Cys-mutant channels were analysed under the control of temperature with the incubation of 5 mM H 2 O 2 (extracellular) or 1 mM DTT (in the pipette) for 15 min . The linear regression lines for the data from WT (black), GGG (blue) and ΔC (blue) channels were indicated. ( c ) Representative current traces of the GGG+T218C mutant channel before (black, left) and after (red, right) the incubation with H 2 O 2 . ( d ) Crosslinking western blot analyses with the oxidation for the Cys-mutant channels. Proteins did not migrate as dimers with reduction (not shown). Full size image The gating cooperativity dependent on the linker structure It has been proposed that the gating movement of one monomeric channel subunit affects the gating of the other subunit within the dimeric unit [16] , [17] , [18] . We observed, in this study, dimerization by the coiled-coil assembly affected the thermosensitive gating. To understand the roles of coiled-coil in the cooperative gating and to know the relationship to the thermosensitive gating, we next analysed the gating cooperativity of channels with mutation in the linker, the GGG mutant and the AAA mutant. We used limiting slope analysis to estimate the effective gating charge in WT and the mutant channels, where the only small amplitude of the H + current is used for analysis with avoiding H + accumulation effects, because the Hv channel gating is sensitive to pH (ref. 32 ). Whole-cell currents were recorded by slow ramp pulse protocols, and reversal potentials, before and after the ramp pulse, were analysed ( Fig. 6a ). Under these conditions, we confirmed that the reversal potentials were not changed after the ramp pulse ( Fig. 6b), and we calculated the chord conductance using the reversal potentials. The value of the effective gating charge (Zδ) in the WT channel was 4.1±0.2 ( n =6), and it was decreased to 2.0±0.03 ( n =5) on deletion of the coiled-coil domain ( Fig. 6c,d ). This twofold Zδ value of the WT channel comparing with the monomeric ΔC channel suggests that two channel subunits gate in a cooperative manner. Introduction of the GGG mutation into the linker segment decreased Zδ to half (2.2±0.03, n =5), whereas the AAA mutation did not affect the Zδ value (4.1±0.1, n =6). Crosslinking assays showed that these two channels express as dimeric channels ( Fig. 4d ). This indicates that dimerization is necessary but not sufficient to establish the gating cooperativity. The stable linker structure is also required for cooperative gating. Cooperative gating of the GGG mutant and the AAA mutant paralleled the result of thermosensitive activation gating ( Figs 4b and 6 ). Zδ values of the channels with mutation in the coiled-coil domain were also analysed. 4R mutation decreased Zδ (2.5±0.1, n =6), whereas the NIN mutation showed an intact gating cooperativity (Zδ=4.2±0.09, n =8). The finding that the channel gating dependent on transmembrane voltage was affected both by the coiled-coil assembly and by the linker mutations suggests that the cytoplasmic coiled-coil domain has mechanical interactions with the transmembrane domain through the linker region. 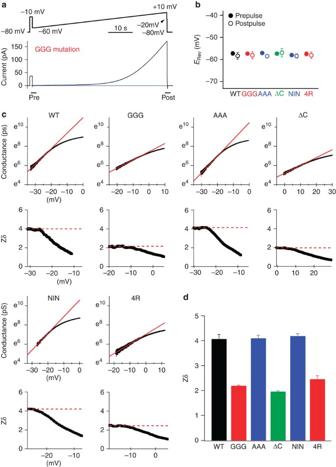Figure 6: The gating cooperativity depends on the linker sequence. (a) A representative H+current through the GGG mutant channel (bottom) in response to a slow ramp pulse from −60 mV to +10 mV (top). Reversal potentials before and after the ramp pulse were measured by step pulses (underlined as 'pre' and 'post'). Because of the variation of the threshold among the constructs, the ramp pulses (1.5 mV s−1) were applied from −50 mV to +40 mV for the ΔC channel, from −60 mV to 0 mV for WT and the AAA mutant channel and from −50 mV to +20 mV for the NIN and the 4R mutant channels, respectively. (b) Reversal potentials (ERev) in WT and the mutant channels. pHi=6 and pHo=7. Symbols depict means and s.e.m. (n=6 in WT,n=5 in GGG,n=6 in AAA,n=5 in ΔC,n=8 in NIN andn=6 in 4R). (c) Representative chord conductance of WT and the mutants (top) and fittings of the slope factor Zδ for different voltages (bottom). The chord conductances were calculated by the prepulseERevand the current amplitude evoked by the ramp pulse. The slope factors were fitted linearly in the marginal conductance range (top and bottom). Thresholds varied among channels (WT=−33±2.0 mV, GGG=−20±1.1 mV, AAA=−29±1.3 mV, ΔC =−3.0±1.3 mV, NIN=−28±1.9 mV and 4R=−19±1.4 mV). (d)The effective gating charge in WT and the mutant channels. Bars depict means and s.e.m. Figure 6: The gating cooperativity depends on the linker sequence. ( a ) A representative H + current through the GGG mutant channel (bottom) in response to a slow ramp pulse from −60 mV to +10 mV (top). Reversal potentials before and after the ramp pulse were measured by step pulses (underlined as 'pre' and 'post'). Because of the variation of the threshold among the constructs, the ramp pulses (1.5 mV s −1 ) were applied from −50 mV to +40 mV for the ΔC channel, from −60 mV to 0 mV for WT and the AAA mutant channel and from −50 mV to +20 mV for the NIN and the 4R mutant channels, respectively. ( b ) Reversal potentials ( E Rev ) in WT and the mutant channels. pHi=6 and pHo=7. Symbols depict means and s.e.m. ( n =6 in WT, n =5 in GGG, n =6 in AAA, n =5 in ΔC, n =8 in NIN and n =6 in 4R). ( c ) Representative chord conductance of WT and the mutants (top) and fittings of the slope factor Zδ for different voltages (bottom). The chord conductances were calculated by the prepulse E Rev and the current amplitude evoked by the ramp pulse. The slope factors were fitted linearly in the marginal conductance range (top and bottom). Thresholds varied among channels (WT=−33±2.0 mV, GGG=−20±1.1 mV, AAA=−29±1.3 mV, ΔC =−3.0±1.3 mV, NIN=−28±1.9 mV and 4R=−19±1.4 mV). ( d )The effective gating charge in WT and the mutant channels. Bars depict means and s.e.m. Full size image Secondary structure analysis of the linker segment To understand the mechanism of the gating regulation by the coiled-coil assembly, the structure information of the linker segment is required. To gain insight into the structure of the linker segment, we expressed and purified the coiled-coil regions, harbouring the linker peptides, and analysed their helix contents by CD spectrum. Measurements of all the coiled-coils CD spectrum revealed minima at 208 and 222 nm ( Fig. 7a ), enabling estimation of the helix contents from the CD spectrum ( Fig. 7b ) [33] . The helix content of the mHv1/VSOP-cc harbouring the original linker peptides (WT-linker) was 86.0%, suggesting that the linker peptides form α-helix. The GGG mutation into the linker decreased the helix content, whereas the AAA mutation retained the high helicity. This suggests that the linker peptide constructs continuous α-helix from the coiled-coil to the transmembrane S4, supporting that the cooperative gating between two subunits is mediated through the coiled-coil assembly. Thermal stabilities of the coiled-coil proteins harbouring the linker peptides are not changed by the mutation ( Fig. 7c ), suggesting that a difference in the temperature-dependent activation between AAA and GGG mutants is caused by the structural difference of the linker region. 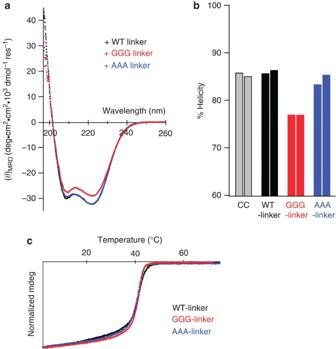Figure 7: Evidence for α-helicity of the linker region by CD. (a) CD spectrum of the mHv1/VSOP-cc harbouring the linker peptides at 4 °C. The amino-acid sequences of the linker region are shown inFig. 4aandSupplementary Fig. S9. (b) Helix contents estimated by CD spectrum. Each two data sets were obtained for the protein constructs. CC is the crystal construct (the mHv1/VSOP-cc protein). Details of the protein constructs analysed are indicated inSupplementary Fig. S9b,f. (c) Melting temperature analysis of the coiled-coil proteins harbouring the linker peptides. Temperature dependence of the CD signal recorded from the coiled-coil proteins harbouring the linker peptides at 222 nm. Figure 7: Evidence for α-helicity of the linker region by CD. ( a ) CD spectrum of the mHv1/VSOP-cc harbouring the linker peptides at 4 °C. The amino-acid sequences of the linker region are shown in Fig. 4a and Supplementary Fig. S9 . ( b ) Helix contents estimated by CD spectrum. Each two data sets were obtained for the protein constructs. CC is the crystal construct (the mHv1/VSOP-cc protein). Details of the protein constructs analysed are indicated in Supplementary Fig. S9b,f . ( c ) Melting temperature analysis of the coiled-coil proteins harbouring the linker peptides. Temperature dependence of the CD signal recorded from the coiled-coil proteins harbouring the linker peptides at 222 nm. Full size image To know the relationships between channel assembly and the function in Hv1/VSOP, we took a multidisciplinary approach, utilizing CD spectroscopy, electrophysiology and X-ray crystallography. We found that the cytoplasmic coiled-coil has key roles both in dimer assembly and gating. Ion channel subunits assemble as multimers to attain adequate functionality. Voltage-gated K + channel subunits assemble into a tetramer to compose the pore in the centre and to attain steep voltage dependence [30] , [34] . Moreover, the assembly of different combinations of pore-forming subunits yields a family of heteromultimeric channels exhibiting functional diversity [25] , [35] , [36] . In the case of the Hv channel, the dimeric coiled-coil assembly regulates the channel activation kinetics in a temperature-dependent manner, such that depolarization-induced increases in H + conductance seems to be optimized in the range of body temperature (cf. WT and ΔC in Fig. 2a,b ). In fact, a Hv channel exhibiting high temperature dependence [37] , [38] is expressed in phagocytes and lymphocytes and contributes to immunological events such as phagocytosis and the antibody production that occur under conditions of local and whole-body fever [3] , [4] , [5] , [6] . The temperature-dependent activation of mHv1/VSOP showed two key features in our study: the temperature dependences for activation (slopes of the channel gating) with the coiled-coil domain deleted ( Fig. 2b ) and mutated ( Fig. 3b ) are virtually identical to those of WT channels; and the temperature dependence of the unfolding of the coiled-coil domain is much steeper ( Fig. 3d ) and occurs over a different temperature range than the temperature-sensitive gating of the channel ( Fig. 3b ). These results imply that the coiled-coil domain does not determine the slope of temperature dependence and that the difference in the activation rate over a range of temperatures is simply due to a difference in the energy of activation. In other words, the higher energetic impact (the higher temperature) is required because of the restriction by the coiled-coil assembly for transition to the channel open state. This was also ascertained in the analysis of the effective charge movement ( Fig. 6 ): the twice valence of the Zδ was observed in WT channel by comparison with ΔC channel. The 4R mutation, which suppressed the coiled-coil assembly and destabilized the thermostability of the gating, reduced Zδ ( Fig. 6c,d ). The results of the effective charge from the GGG/AAA linker mutant channels also well-matched to those in the analysis on the temperature-dependent activation ( Figs 4 and 6 ), suggesting that the modulation of the temperature-dependent activation by the coiled-coil assembly lies in the same biophysical principle to the cooperative gating of the channel. Thus, the gating cooperativity of the mHv1/VSOP channel depends on the structural base consisting of the coiled-coil domain and the linker domain, and the coiled-coil assembly adjusts the range of temperature by elevating the energy of activation for the channel opening. Effect of the pre-heating at high temperature on activation kinetics was reversible ( Supplementary Fig. S3c ), and this seems inconsistent with the results of the CD spectrum ( Fig. 3d ). However, this is most likely caused by the difference of physical condition of the coiled-coil; that is, the coiled-coil domain below the close unit of two transmembrane domains may acquire a reversible dissociation, whereas the purified protein hardly finds assembly partner in solution. Live monitoring of the coiled-coil domain behaviour during the channel gating, by some techniques, will merit further research. Schematic illustrations of gating in the WT and the mutant channels are summarized ( Fig. 8a-c ). The stabilizing regulation of the temperature-dependent activation by the coiled-coil was observed in the WT channel ( Fig. 8a , red arrow), while it conversely disappeared and the temperature threshold of the activation kinetics was set lower in the 4R and GGG channels ( Fig. 8b,c , red broken arrow). The gating cooperativity was also reduced in the 4R and GGG mutation . These are caused by the unstable dimerization of the 4R coiled-coil and by the loose connection via the GGG linker ( Fig. 8b,c ). Phenotypes of the AAA channel in the temperature-dependent activation and the cooperative gating were the same to those of the WT channel. The ΔC channel does not have a coiled-coil domain and the gating partner, and therefore regulation of the temperature dependent activation was destabilized and the cooperative gating disappeared. Thus, rigid structure of the linker region enables to mediate the stability of the coiled-coil to the transmembrane domain, and to mediate the cooperative gating within the dimer. Considering the mechanical interaction between two channel subunits, a certain level of physical intersubunit contact between transmembrane regions within a dimer has been reported [9] , [17] . These make it plausible that two transmembrane regions in close proximity in a dimer physically interact with one another, and the coiled-coil domain facilitates the close positioning of the two transmembrane regions ( Supplementary Fig. S7a ). However, this idea is inconsistent with our finding that GGG mutation at the linker region eliminated the WT gating phenotype, but retained the dimeric assembly ( Fig. 4b,d ). The phenotypes of GGG mutant were unchanged in the condition in which the cytoplasmic ends of two S4 helixes were crosslinked by disulfide bonding ( Fig. 5 ). Our results provide an alternative model in which cooperative gating of the two channel units is mediated by mechanical interaction via the cytoplasmic coiled-coil ( Supplementary Fig. S7b ). The linker structure is α-helix from the results with the CD spectrometry ( Fig. 7 ), suggesting that the force transmission takes place along a continuous α-helix consisting of the S4 and the coiled-coil strands ( Fig. 8a ; Supplementary Fig. S7b ). The coiled-coil structure is thus a suitable cytoplasmic domain that accomplishes both subunit assembly and gating modulation. 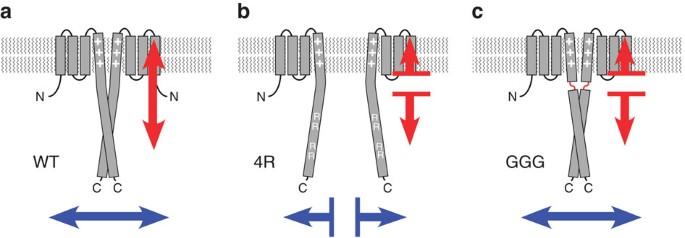Figure 8: Schematic drawings of the gating in a dimeric Hv channel. (a) Schematic drawings of the regulation of temperature-dependent gating by the cooperation of coiled-coil region (red arrow) and the dimerization of Hv protomers by coiled-coil (blue arrow) in the WT (or the AAA mutant) channel. Rigid structure of the linker region and the stable coiled-coil mediate the thermostability of channel activation based on the cooperative gating within the dimer . (b) Model of the 4R mutant channel. The channel dimerization is disrupted due to the instability of the coiled-coil assembly (broken blue arrow) that results in instability, the lower threshold, of the temperature-dependent activation (red broken arrow). (c) Model of the GGG mutant channel. Although the channel is dimerized (blue arrow), the thermostability of channel activation is not mediated by the coiled-coil domain (red broken arrow) due to the loose connection by the GGG linker. Figure 8: Schematic drawings of the gating in a dimeric Hv channel. ( a ) Schematic drawings of the regulation of temperature-dependent gating by the cooperation of coiled-coil region (red arrow) and the dimerization of Hv protomers by coiled-coil (blue arrow) in the WT (or the AAA mutant) channel. Rigid structure of the linker region and the stable coiled-coil mediate the thermostability of channel activation based on the cooperative gating within the dimer . ( b ) Model of the 4R mutant channel. The channel dimerization is disrupted due to the instability of the coiled-coil assembly (broken blue arrow) that results in instability, the lower threshold, of the temperature-dependent activation (red broken arrow). ( c ) Model of the GGG mutant channel. Although the channel is dimerized (blue arrow), the thermostability of channel activation is not mediated by the coiled-coil domain (red broken arrow) due to the loose connection by the GGG linker. Full size image The coiled-coil design of the Hv channel is unique in that a hydrophilic residue, N231, is present within the hydrophobic core alignment. As seen in the flipped geometry of the side chains in comparison with the hHv1/VSOP coiled-coil [19] ( Fig. 1c ), N231 could contribute to increase flexibility of the coiled-coil. NIN mutation increased the thermostability—that is, the fold was reversible after melting ( Fig. 3d ). Correspondingly, the higher temperature was required to evoke an activation of the NIN mutant channel ( Fig. 3b ). This seemingly unusual hydrophilic N231 core, conserved among all species of Hv channel ( Fig. 1a ), may be installed among the hydrophobic residues to adjust the stability or generate mobility within the coiled-coil domain during channel gating, enabling proper regulation of channel activation ( Fig. 3a,b ). Findings derived from the study of Hv channels, a minimal voltage-gated channel, may offer principles common to other larger and more complex ion channels; force transmission between the cytoplasmic domain and the gate within the transmembrane region may also occur in other ion channels in which gating modulators interact with a region adjacent to the transmembrane gate [39] , [40] , [41] , [42] , [43] . Cloning and the construction design We used a mouse Hv channel clone (mHv1/VSOP) [1] for all experiments in this study. In the experiments of protein biochemistry ( Figs 1c and 7 ), DNA corresponding to the mHv1/VSOP coiled-coil domain (residues 220–269) was amplified by PCR and ligated into a pET28 (Novagen)-derived vector, pET28HMT [44] , kindly given by Dr Daniel L. Minor Jr (UCSF, USA). In the experiments of electrophysiology ( Figs 2 , 3 , 4 , 5 , 6 ), the complementary DNAs for WT and mutant mHv1/VSOP channels were subcloned into the pIRES-EGFP expression vector (Clontech). In the recordings of the concatenated channel, two subunits were linked with a flexible 19-amino-acid linker, GGSGGSGGSGSGGSGGSGG, as a tandem channel ( Fig. 4a ). In the crosslinking assay by disulfide-bond, the double-point mutant of mHv1/VSOP, C103S and C245S, was used as a template, where two native Cys residues were mutated to prevent intrinsic disulfide bondings ( Fig. 5 ). The constructs used are summarized in Supplementary Fig. S9 . Crosslinking assay HEK293T cells were used as the expression host for mHv1/VSOP WT and mutant channels. In the amine-reactive crosslinking ( Figs 1b and 4d ), cells were treated by DSS and the reaction was quenched with 100 mM Tris HCl (pH 8.0). In the crosslinking analyses by disulfide bond ( Fig. 5d ), cells were lysed with 1% dodecyl maltoside, and, then, the protein solution was oxidized by Cu–P (mixture of 330 μM CuSO 4 and 1 mM O-phenanthroline) for 20 min. The Cu–P reaction was quenched with 5 mM N-ethylmaleimide and 50 mM EDTA. Proteins were separated on 12.5% SDS–PAGE under reducing conditions and electrophoretically transferred to Immobilon-P (Millipore). A polyclonal rabbit anti-mHv1/VSOP antibody generated against the amino acids Met 1 -Ala 72 in the N terminus of mHv1/VSOP was used for detection [45] . Horseradish peroxidase-conjugated donkey anti-rabbit IgG (Amersham Pharmacia) was used as the secondary antibody. Protein expression and purification Proteins were expressed in Escherichia coli. (BL21(DE3)pLysS) grown in 2YT media at 37 °C and induced with 0.4 mM isopropyl-β-D-thiogalactoside for 4 h. Cells were harvested by centrifugation, and cell pellets were lysed by sonication in lysis buffer (10 mM K 2 HPO 4 pH 7.3, 250 mM KCl, 1 mM EDTA, 5 mM β-ME, 1 mM PMSF). The soluble fraction, which contained the hexahistidine-maltose-binding protein tag, was applied to a 20-ml HisPrep FF (GE Healthcare) nickel-charged column, and eluted by 500 mM imidazole on an ÄKTA-purifier system (GE Healthcare). The proteins were then applied to a 75-ml amylose (New England Biolabs) column, and eluted by 10 mM maltose, after which the maltose was removed on a 53-ml HiPrep desalting column (GE Healthcare). The affinity tag was then cleaved with TEV protease [46] (~300 μM for 24 h, at 4 °C). Coiled-coil proteins were collected in the flow-through from the Hisprep nickel column, and were further purified by Superdex75 gel-filtration column (GE Healthcare). The protein concentration was determined by absorbance (BCA Protein Assay Kit, Pierce), and the solution of purified mHv1/VSOP coiled-coil protein (mHv1/VSOP-cc) was used for the crystallization step. Crystallography mHv1/VSOP-cc crystals were obtained at 10 °C using hanging-drop vapour diffusion. The crystals grew from mixtures of 1 μl of protein solution (5 mg ml −1 protein dissolved in 150 mM KCl, 5 mM Hepes (pH 7.3)) and 1 μl of reservoir solution containing 2% v/v Tacsimate (pH 7.0), 0.1 M imidazole (pH 7.0), 8% w/v PEG3350, and 5% v/v 2-Propanol (PEGRx-2 #26, Hampton) ( Fig. 1c ). Diffraction data were collected using 20% PEG200 cryoprotectant at BL44XU SPring-8 (Hyogo) equipped with a MX-225HE CCD detector (Rayonix). The mHv1/VSOP-cc crystals belonged to the P 2 1 2 1 2 1 space group and diffracted X-rays to 1.45 Å. Data were processed using HKL2000 (HKL Research). The primary structure was solved by molecular replacement with Phaser [47] using a dimeric coiled-coil template (1D7M), and an initial structural model was built using the program Arp/Warp [48] . Model building was done in Coot [49] . A resultant model was refined using REFMAC5 (ref. 50 with the inclusion of TLS parameters throughout refinement (PDB accession code 3VMX ) ( Supplementary Table S1 ). The structural comparison between mHv1/VSOP coiled-coil (222–262) and hHv1/VSOP coiled-coil (226–266; PDB accession code 3A2A ) was carried out using lsqkab in CCP4 suite, and the r.m.s. deviation calculated was obtained. CD spectroscopy Protein solution, composed of 50-μM purified mHv1/VSOP coiled-coil protein in buffer containing 150 mM KCl, 1 mM DTT and 10 mM K 2 HPO 4 (pH 7.3), was analysed using an J-715 spectropolarimeter (JASCO) equipped with a peltier device. The protein concentration was adjusted by absorbance using a measuring template, the protein construct harbouring Trp for the sedimentation analysis, whose concentration was determined by absorbance at 280 nm (refs 51 , 52 ). The protein constructs analysed were summarized ( Supplementary Fig. S9f ). Wavelength scans from 260 to 190 nm were taken at 4 °C, using a 1-mm path length cuvette. Thermal stability was assessed by monitoring [θ] 222 every 0.2 °C from 4 to 85 °C, using a 1-°C min −1 temperature gradient. Molar ellipticity per residue of the buffer-subtracted CD spectrum was calculated as a function of concentration, path length, and number of residues per monomer: where [ θ ] MRD is the molar ellipticity per residue in deg·cm 2 (dmol·res) −1 , θ is the experimental ellipticity in millidegrees, M is the molecular mass of the protein, c is the protein concentration in μM, l is the cuvette path length in mm, and NR is the number of residues in the protein. The per cent helicity was estimated by: where [ θ ] 222 is the experimental molar ellipticity per residue at 222 nm, is the molar ellipticity for a helix of infinite length at 222 nm (that is, 39,500 deg·cm 2 dmol −1 ), i is the number of helices, κ is a wavelength-specific constant with a value of 2.57 at 222 nm, and N is the number of residues in the protein [33] . Electrophysiology The cDNAs for WT and mutant mHv1/VSOP channels were transfected into HEK293T cells. The cells were then cultured for 24 h in DMEM supplemented with 10% bovine calf serum. Electrophysiological recordings were carried out 4–16 h after reseeding, which corresponds to 18–30 h after transfection. A coverslip with HEK293T cells was placed in a recording chamber containing bath solution (see below) on the stage of an inverted fluorescence microscope (IX71, Olympus), and the transfected cells were identified by the fluorescent signal from the green fluorescent protein. Macroscopic currents were then recorded in the whole-cell clamp configuration using an Axopatch-200B amplifier (Molecular Devices). The pipette resistance in the solution was 3–5 MΩ. Sixty-to-eighty per cent of the voltage error due to the series resistance was compensated by a circuit in the amplifier. The recorded currents were low-pass filtered at 1 kHz using a 4-pole Bessel filter circuit built into the amplifier. The external solution contained 75 mM N-methyl- D -glucamine (NMDG), 1 mM CaCl 2 , 1 mM MgCl 2 , 10 mM glucose, and 180 mM Hepes (pH 7.0). The pipette solution contained 65 mM NMDG, 3 mM MgCl 2 , 1 mM EGTA, and 183 mM Hepes (pH 7.0). For analysing the effective gating charge ( Fig. 6 ), the pipette solution contained 75 mM NMDG, 1 mM MgCl 2 , 1 mM EGTA, 70 mM glucose, and 110 mM MES (pH 6.0). The recording temperature was controlled (15–45 °C) by adding heated or cold external solution to the external solution. Data were analysed using Clampfit (Axon Instruments) and Igor Pro (WaveMetrics) software. The activation time constant shown in Figs 2 , 3 , 4 , 5 and Supplementary Figs S3–S4 was obtained by fitting the activation phase of the outward currents on depolarization at 100 mV from the onset of the step pulse to the pulse end. Various lengths of pulse time, 500 ms, 625 ms, 1, 1.25, 1.5, 2, 3 and 5 s were used to fit the activation phases properly by single exponential function, and an inverse logarithm (Log(1/ τ )) of the activation time constant ( τ ) was calculated and plotted versus temperature ( Figs 2 , 3 , 4 , 5 and Supplementary Figs S3-S4 ). Size-exclusion chromatography For the isolated HMT-tagged mHv1/VSOP coiled-coil, 100 μl of 500 μM protein in buffer containing 250 mM KCl, 10 mM Tris (pH 7.3) were passed through a Superdex200 HR 10/30 column (GE Healthcare) equilibrated with the same buffer on an ÄKTA-purifier system (GE Healthcare) at 4 °C (refs 25 , 53 ). Elutes were monitored at 280 nm over a flow rate of 0.5 ml min −1 . Each column was calibrated using six standard protein molecular mass markers ( Supplementary Fig. S8 ). Elution volumes from three runs were averaged. In the statistical analysis, mean±s.e.m. was indicated unless otherwise noted. Equilibrium sedimentation Equilibrium sedimentation experiments were performed at 4 °C in a Beckman Optima XL-A analytical ultracentrifuge (Beckman Coulter) ( Supplementary Fig. S1a ). The mHv1/VSOP-cc-GGWS was dissolved to a concentration of 40 μM in 150 mM KCl, 1 mM DTT, 10 mM K 2 HPO 4 (pH 7.3), and the equilibrium distribution was measured based on the absorbance at 275 nm as a function of the radial distance at 25,000 r.p.m., at 4 °C. The molecular mass and residuals were calculated, as described previously [25] , [54] . Accession codes: The structure coordinates for the mHv1/VSOP coiled-coil have been deposited in the Protein Data Bank under code 3VMX . How to cite this article: Fujiwara Y. et al . The cytoplasmic coiled-coil mediates cooperative gating temperature sensitivity in the voltage-gated H + channel Hv1. Nat. Commun. 3:816 doi: 10.1038/ncomms1823 (2012).